Real-time single-molecule co-immunoprecipitation analyses reveal cancer-specific Ras signalling dynamics Co-immunoprecipitation (co-IP) has become a standard technique, but its protein-band output provides only static, qualitative information about protein–protein interactions. Here we demonstrate a real-time single-molecule co-IP technique that generates real-time videos of individual protein–protein interactions as they occur in unpurified cell extracts. By analysing single Ras–Raf interactions with a 50-ms time resolution, we have observed transient intermediates of the protein–protein interaction and determined all the essential kinetic rates. Using this technique, we have quantified the active fraction of native Ras proteins in xenograft tumours, normal tissue and cancer cell lines. We demonstrate that the oncogenic Ras mutations selectively increase the active-Ras fraction by one order of magnitude, without affecting total Ras levels or single-molecule signalling kinetics. Our approach allows us to probe the previously hidden, dynamic aspects of weak protein–protein interactions. It also suggests a path forward towards precision molecular diagnostics at the protein–protein interaction level. Cell signalling, first initiated at the cell membrane, propagates through the cytoplasm to finally regulate patterns of gene expression deep inside the nucleus. This process, which is mediated by a cascade of generally weak and transient protein–protein interactions, allows the cell to adapt rapidly to changing environmental conditions. To study such protein–protein interactions, biologists currently depend heavily on co-immunoprecipitation (co-IP) followed by a western blot. In these techniques, a protein mixture captured by bait proteins in a pull-down is separated by electrophoresis and subsequently stained for specific protein components with antibodies [1] . Despite the enormous contribution the co-IP and western blot techniques have made to modern molecular biology, these methods have an inherent limitation as qualitative methods. Although western blots can produce a narrow protein band, the intensity of which correlates with the amount of the protein it contains, it is often difficult to calibrate the band intensity and determine the true molar concentration of any given protein. Furthermore, if the proteins in question were captured using co-IP, the band intensity is also used to assess the strength of a protein–protein interaction. Such bands, however, contain less quantitative information than straight western bands, because they have lost all information regarding the kinetic details of the protein–protein interactions. Thus, the abilities to precisely quantify the contextual concentration of specific proteins and dissect the kinetics of their interactions are the critical knowledge gaps that the traditional western blot and co-IP techniques cannot fill. Recently, a single-molecule pull-down technique was reported, in which tiny amounts of a target protein from cell extracts could be selectively captured on a surface using polymer cushions and biotinylated antibodies [2] . This report suggests the potential contributions single-molecule fluorescence spectroscopy could make to the traditional molecular biology techniques. Until now, single-molecule pull-down techniques [2] , [3] have only been capable of addressing immobilized protein complexes that are stable for minutes to hours. The subunit composition of these static protein complexes has been determined by counting the number of photobleaching steps, which is done after the removal of the original cell extracts. This is essentially doing the conventional co-IP and then using single-molecule fluorescence spectroscopy to visualize the results instead of using a traditional western blot [4] . In this work, we demonstrate real-time imaging of a single-molecule co-IP preparation. By maintaining unpurified cell extracts in the imaging chamber, the protein–protein interactions can be recorded in real time at a 50-ms time resolution. In other words, we are imaging the co-IP process itself as it happens, which is the technical arena that the conventional co-IP technique cannot address ( Supplementary Fig. S1 ). This real-time single-molecule co-IP technique allows us to probe the rich and dynamic, but previously hidden, aspects of weak protein–protein interactions. We have used our real-time single-molecule co-IP analyses to quantitatively study native cell signalling proteins. We determined, for the first time, the fraction of the signalling proteins that were actively binding to downstream targets. In the case of Ras signalling, we observed that oncogenic Ras mutations increase this active fraction of Ras proteins, without affecting the Ras expression level or single-molecule signalling kinetics. The approaches described here suggest a general strategy for characterizing specific cancers at the level of their protein–protein interactions. Real-time imaging of single-molecule co-IP We first show that the kinetics of a protein–protein interaction can be measured in cell extracts at the single-molecule level ( Fig. 1 ). As a model interaction in a cell signalling pathway, we chose the interaction between Ras and Raf, which is the initial step of the conserved MAPK pathway that is hyper-activated in many human cancers [5] , [6] , [7] . We used the Ras-binding domain of cRaf (cRaf RBD ) and a version of HRas containing a single-point mutation, Q61L, which makes it constitutively active [6] , [8] , [9] , [10] , [11] , [12] . Live cell imaging of HeLa cells co-expressing these two proteins showed a high level of co-localization ( Fig. 1a and Supplementary Fig. S2 ). We were able to direct this co-localization with rapamycin-triggered translocation of HRas to the plasma membrane [13] , which resulted in concurrent localization of cRaf RBD to the same spots. The conventional co-IP also produced a clear western band, indicating a selective protein–protein interaction between constitutively active HRas and cRaf RBD ( Fig. 1b , left). However, we found out that this apparently clear protein band contained only less than 5% of the entire prey proteins, suggesting that the prey proteins might not be stably bound to baits but removed to the flow-through portion through washing processes ( Fig. 1b , right and Supplementary Fig. S3 ). We further note that both of the live cell imaging and co-IP approaches cannot dissect the real kinetics of this perhaps weak, transient protein–protein interaction. 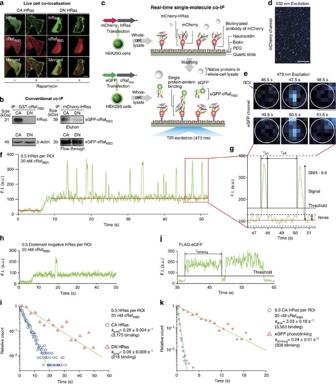Figure 1: Real-time single-molecule co-IP imaging. (a) Live cell co-localization study for the HRas–cRafRBDinteraction. Protein–protein interactions between HRas and cRafRBDwere assessed by observing the translocation of cRafRBDto the plasma membrane along with HRas. CA and DN denote the constitutively active and dominant negative forms of HRas, respectively. Scale bar, 10 μm. (b) Conventional co-IP data for the HRas–cRafRBDinteraction. For the co-IP analyses, GST-cRafRBD(left) and mCherry-HRas proteins (right) were used, respectively, as the baits immobilized on beads. (c) Schematic of the real-time single-molecule co-IP. (d) TIRF image of immobilized mCherry-HRas on surface. Scale bar, 10 μm. (e) Successive frames from real-time imaging of single-molecule co-IP. The real-time trace of these binding events is shown infand marked with a red square. Scale bar, 1 μm. (f,g) Exemplary real-time traces from the real-time single-molecule co-IP imaging. The signal mainly consists of a diffuse background fluorescence super-imposed with a sequence of fluorescence spikes. (h) A negative control experiment with surface-immobilized DN HRas (S17N). (i) Distributionkbindfor the experiment inf. Relevant kinetic rates were determined using a single-exponential curve fit (solid lines). (j) A second negative control experiment with surface-immobilized FLAG-eGFP. (k) Distribution ofkdissfor the experiment inf. Andkblinkingfor the experiment inj. Relevant kinetic rates were determined using a single-exponential curve fit (solid lines). Error bars denote standard error (s.e.;n>200). Figure 1: Real-time single-molecule co-IP imaging. ( a ) Live cell co-localization study for the HRas–cRaf RBD interaction. Protein–protein interactions between HRas and cRaf RBD were assessed by observing the translocation of cRaf RBD to the plasma membrane along with HRas. CA and DN denote the constitutively active and dominant negative forms of HRas, respectively. Scale bar, 10 μm. ( b ) Conventional co-IP data for the HRas–cRaf RBD interaction. For the co-IP analyses, GST-cRaf RBD (left) and mCherry-HRas proteins (right) were used, respectively, as the baits immobilized on beads. ( c ) Schematic of the real-time single-molecule co-IP. ( d ) TIRF image of immobilized mCherry-HRas on surface. Scale bar, 10 μm. ( e ) Successive frames from real-time imaging of single-molecule co-IP. The real-time trace of these binding events is shown in f and marked with a red square. Scale bar, 1 μm. ( f , g ) Exemplary real-time traces from the real-time single-molecule co-IP imaging. The signal mainly consists of a diffuse background fluorescence super-imposed with a sequence of fluorescence spikes. ( h ) A negative control experiment with surface-immobilized DN HRas (S17N). ( i ) Distribution k bind for the experiment in f . Relevant kinetic rates were determined using a single-exponential curve fit (solid lines). ( j ) A second negative control experiment with surface-immobilized FLAG-eGFP. ( k ) Distribution of k diss for the experiment in f . And k blinking for the experiment in j . Relevant kinetic rates were determined using a single-exponential curve fit (solid lines). Error bars denote standard error (s.e. ; n >200). Full size image To visualize the HRas–cRaf RBD interaction in real time at the single-molecule level, we fused the HRas gene with the red fluorescent protein mCherry and we fused cRaf RBD with enhanced green fluorescent protein (eGFP; Fig. 1c ). We expressed each protein in a separate group of HEK293 cells. We used the strategy of single-molecule pull-down to immobilize mCherry-HRas on the surface [2] , [3] ( Fig. 1c ). We then injected the second whole-cell lysate containing eGFP-cRaf RBD onto the mCherry-HRas immobilized surface as in a conventional co-IP ( Fig. 1c ). We used a total internal reflection (TIR) microscope to generate an evanescent electric field that selectively excited eGFP-cRaf RBD s that came within 100 nm of the surface. To observe weak protein–protein interactions, single eGFP-cRaf RBD arrivals at the surface were monitored in real time with the second whole-cell lysate maintained in the chamber ( Fig. 1c ). Figure 1f shows a typical real-time trace of this single-molecule co-IP preparation. Each trace was produced by integrating the fluorescence signal over a circular region of interest (ROI) with an area of 1.1 μm 2 ( Fig. 1e ). We controlled the surface density of mCherry-HRas to maintain an average of 0.5 HRas molecule per ROI ( Supplementary Fig. S4 ). We also used Gaussian filtering during signal integration and a stringent threshold for signal detection to ensure that the real-time traces reported the binding events of single-HRas proteins ( Fig. 1g and Supplementary Fig. S5 ). Each real-time trace clearly consists of two parts: a background fluorescence and individual fluorescence spikes. Each eGFP-cRaf RBD molecule, moving according to Brownian motion, should spend less than 50 μs per visit to the TIR excitation layer. As 50 μs is three orders of magnitude shorter than the time resolution of our imaging apparatus (50 ms), the Brownian motion of many eGFP-cRaf RBD molecules produce a constant level for background fluorescence. The individual fluorescence spikes, on the other hand, indicate that a single eGFP-cRaf RBD has interacted with a molecule on the surface long enough to survive the 50 ms signal integration. We next analysed the essential kinetics of this protein–protein interaction by analysing τ off , the time between binding events, and τ on , the duration of a single-binding event ( Fig. 1g ). Fitting single exponential equations to the τ off and τ on distributions gives the kinetic rates of k bind and k diss , respectively. To ensure that the fluorescence spikes are indeed the result of a specific HRas–cRaf RBD interaction, we performed the same eGFP-cRaf RBD binding experiment with surface-immobilized dominant negative HRas (S17N), which has a reduced affinity to GTP [14] , [15] . With the dominant negative form, the fluorescence spike frequency ( k bind ) was seriously diminished ( Fig. 1h ). This negative control proves that the fluorescence spikes are neither artefacts of simple eGFP-cRaf RBD surface adsorption nor are they due to surface immobilization of other proteins with spurious eGFP–cRaf RBD interactions. Instead, these fluorescence spike traces faithfully report the HRas-cRaf RBD binding events. It is also remarkable that the duration of a single-binding event typically lasts only a few hundred ms ( Fig. 1f ). We studied the blinking dynamics of FLAG-eGFP [16] immobilized to a surface with an anti-FLAG antibody ( Fig. 1j ). Photo-blinking of FLAG-eGFP occurs on average every few seconds, giving a kinetic rate smaller than 0.3 s −1 , and this eGFP photoblinking rate is one order of magnitude slower than the k diss we measured ( Fig. 1k ). Moreover, we revalidated all the single-molecule kinetic rates of k bind and k diss using a co-localization criterion that required co-location of fluorescence signals from the mCherry-HRas and eGFP-cRaf RBD proteins ( Supplementary Fig. S6 ). Thus, the HRas–cRaf RBD interaction must indeed have rapid turnover, a few times per second [11] , [12] . Visualization of encounter complexes in Ras-Raf interaction Detailed analysis of the HRas-cRaf RBD binding frequency ( k bind ) indicates the existence of fast pre-equilibrating encounter complexes [17] , [18] , [19] , [20] , [21] , which are loose protein–protein interaction intermediates that should be populated before formation of the final HRas–cRaf RBD complex ( Fig. 2 ). When we increased the concentration of eGFP-cRaf RBD from 5 to 50 nM, the k bind showed a parabolic increase ( Fig. 2a ), which can be best fitted to the equation of with a Hill coefficient ( n ) of 1.1 ( [22] , [23] ), a dissociation constant ( K 1 ) of 43 nM for encounter complex formation, and a κ on of 2.16 s −1 nM −1 , which is the kinetic rate of forming the final bound state from an encounter complex ( Supplementary Methods and Supplementary Fig. S7 ). k diss , on the other hand, is largely constant for the eGFP-cRaf RBD concentrations we studied ( Fig. 2b ). These kinetic rates measured with our real-time single-molecule co-IP are closely consistent with previous reports using bulk biochemical assays ( Supplementary Table S1 ). One note is we have assumed one predominant conformation for the final HRas–cRaf RBD complex. Although our assumption is corroborated by the unimodal distributions of the fluorescence spike intensity ( Supplementary Fig. S8 ), we cannot completely rule out the possibility that there are multiple conformations for the HRas–cRaf RBD complex with multiple pathways leading to them. 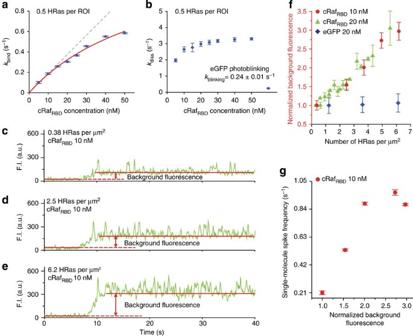Figure 2: Single-molecule kinetic analysis of the HRas–cRafRBDinteraction. (a)kbindas a function of the cRafRBDconcentration. A linear increase inkbindis shown as a comparison. (b)kdissas a function of the cRafRBDconcentration.kblinkingfrom the experiment inFig. 1jis shown as a comparison. Error bars denote s.e. (n>180). (c–e) Real-time traces of HRas–cRafRBDinteraction. Note that the background fluorescence increases with the surface HRas density. We used the same prey concentration of [cRafRBD]=10 nM. (f) Background fluorescence increase as a function of the surface HRas density. Three data sets, obtained with 10 nM (red circles), 20 nM (green triangles) eGFP-cRafRBDand 20 nM recombinant eGFP (blue diamonds), are normalized by the corresponding background fluorescence level measured at a low surface Ras density of 0.38 HRas per μm2. Error bars denote s.d. (n>100). (g) Single-molecule spike frequency as a function of background fluorescence. The data set obtained with 10 nM eGFP-cRafRBDis used. Error bars denote s.e. (n>100). Figure 2: Single-molecule kinetic analysis of the HRas–cRaf RBD interaction. ( a ) k bind as a function of the cRaf RBD concentration. A linear increase in k bind is shown as a comparison. ( b ) k diss as a function of the cRaf RBD concentration. k blinking from the experiment in Fig. 1j is shown as a comparison. Error bars denote s.e. ( n >180). ( c – e ) Real-time traces of HRas–cRaf RBD interaction. Note that the background fluorescence increases with the surface HRas density. We used the same prey concentration of [cRaf RBD ]=10 nM. ( f ) Background fluorescence increase as a function of the surface HRas density. Three data sets, obtained with 10 nM (red circles), 20 nM (green triangles) eGFP-cRaf RBD and 20 nM recombinant eGFP (blue diamonds), are normalized by the corresponding background fluorescence level measured at a low surface Ras density of 0.38 HRas per μm 2 . Error bars denote s.d. ( n >100). ( g ) Single-molecule spike frequency as a function of background fluorescence. The data set obtained with 10 nM eGFP-cRaf RBD is used. Error bars denote s.e. ( n >100). Full size image Remarkably, we can visualize the encounter complexes by varying the surface density of HRas. If the background fluorescence is a simple product of the Brownian motion of eGFP-cRaf RBD , it would depend solely on the bulk cRaf RBD concentration. However, the background fluorescence steeply increases with the surface density of HRas even though the cRaf RBD concentrations are kept constant ( Fig. 2c–f ). At a high Ras density of 6.4 HRas per μm 2 , the total background fluorescence becomes three times as high as that observed at 0.38 HRas per μm 2 ( Fig. 2c ). Our numerical simulation shows that the presence of parallel binding processes in a given ROI can only account for less than 5% of the observed increase ( Supplementary Fig. S9 ). Moreover, when the prey proteins were changed to recombinant eGFPs, which did not interact with surface-immobilized HRas proteins, their background fluorescence was essentially invariant in the HRas density range we studied ( Fig. 2f , blue diamonds). Thus, as we have a dense population of active HRas on the surface, there seems to indeed be more eGFP-cRaf RBD molecules lingering above the surface than would be expected by pure Brownian diffusion. These encounter complexes arise from fast pre-equilibrating interactions between HRas and cRaf RBD proteins [24] , of which dynamics is beyond our temporal resolution. We next questioned whether the encounter complexes indeed serve as substrates for the final HRas–cRaf RBD complex. To this end, we assessed the frequency of fluorescence spikes generated by a single surface-immobilized HRas protein. We have reasoned that if the encounter complexes are true on pathway intermediates for the final Ras–Raf complex, the single-molecule spike frequency should grow with the increasing background fluorescence in spite of the same bulk cRaf RBD concentration. To obtain the single-molecule spike frequency in HRas-dense environments, we measured k bind using a smaller 3 by 3 pixel ROI (0.18 μm 2 ) and divided the measured k bind value by the average number of HRas in each 3 by 3 pixel ROI ( Supplementary Fig. S10 ). By and large, this single-molecule spike frequency increased with the background fluorescence ( Fig. 2g , 10 nM eGFP-cRaf RBD used). Our observation suggests that the concentrated downstream proteins in the form of encounter complexes lead to formation of the Ras–Raf complex with an increased frequency. Single-molecule co-IP analysis of signalling proteins in cancers We have thus far demonstrated the real-time measurement of protein–protein interaction kinetics during single-molecule co-IP. In these experiments, however, the bait and prey proteins are fused to fluorescent protein tags, posing the question of whether we can extend this technique to native proteins. To this end, we expressed mutated HRas (G12V) in a non-tumorigenic human breast epithelial cell line (MCF10A) to transform them into cancerous cells [25] ( Fig. 3a ). These transformed cells, which showed serum-free growth ( Supplementary Fig. S11 ), formed tumours when injected into the mammary fat pad of immunocompromised mice ( Fig. 3b ). Tumour tissues were obtained 17 days after the xenograft, and control tissues were prepared from the same parts of untreated nude mice. 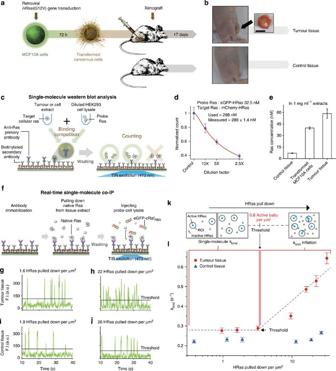Figure 3: Quantitative characterization of signalling proteins in tumour tissue. (a,b) Transformation of MCF10A cells into cancerous cells by retroviralHRas(G12V) transduction. This single-point mutation is known to make HRas constitutively active. Injecting cancerous cells to mammary pad of nude mice leads to tumour formation. Scale bar, 5 mm. (c) Schematic of single-molecule western blot analysis. Competition between cellular and probe Ras for binding to the primary antibody reduces the number of probe Ras specifically bound to the surface, which consequently reduces the number of fluorescent spots. Note that as each primary antibody binds to two Ras proteins, one fluorescent spot disappears when both of two light-chain arms are occupied by cellular Ras. (d) Prototypical single-molecule western blot measurement. 298 nM mCherry-HRas was used as target protein. With 32.5 nM eGFP-HRas as the probe, the target protein concentration was measured to be 288±1.4 nM. Error bar denotes s.d. (n=20). (e) Ras expression levels measured through the process of tumorigenesis froma,b. Error bars denote s.d. (n=20). (f) Schematic of real-time co-IP imaging for native HRas. (g–j) Real-time traces of co-IP imaging. The HRas concentrations used for pull down are 3.0 (g), 41.3 (h), 3.5 (i) and 49 nM (j). The frequency of fluorescence spikes was significantly increased for the cancer tissue extract when HRas pull-down was increased from 1.6 to 22 HRas per μm2(gversush). This was not observed with the control tissue extract (iversusj). (k) Schematic ofkbindinflation. Under sparse conditions of active baits on surface, a constant, single-moleculekbindis obtained even when the surface pull-down of baits is increased (left two panels). However, past the threshold at 0.6 active baits per μm2, more than one baits are present per ROI on average. These multiple baits have the effect of increasingkbindmeasured from each ROI (right panel). (l)kbindas a function of HRas pull-down. Error bars denote s.e. (n>180). Figure 3: Quantitative characterization of signalling proteins in tumour tissue. ( a , b ) Transformation of MCF10A cells into cancerous cells by retroviral HRas (G12V) transduction. This single-point mutation is known to make HRas constitutively active. Injecting cancerous cells to mammary pad of nude mice leads to tumour formation. Scale bar, 5 mm. ( c ) Schematic of single-molecule western blot analysis. Competition between cellular and probe Ras for binding to the primary antibody reduces the number of probe Ras specifically bound to the surface, which consequently reduces the number of fluorescent spots. Note that as each primary antibody binds to two Ras proteins, one fluorescent spot disappears when both of two light-chain arms are occupied by cellular Ras. ( d ) Prototypical single-molecule western blot measurement. 298 nM mCherry-HRas was used as target protein. With 32.5 nM eGFP-HRas as the probe, the target protein concentration was measured to be 288±1.4 nM. Error bar denotes s.d. ( n =20). ( e ) Ras expression levels measured through the process of tumorigenesis from a , b . Error bars denote s.d. ( n =20). ( f ) Schematic of real-time co-IP imaging for native HRas. ( g – j ) Real-time traces of co-IP imaging. The HRas concentrations used for pull down are 3.0 ( g ), 41.3 ( h ), 3.5 ( i ) and 49 nM ( j ). The frequency of fluorescence spikes was significantly increased for the cancer tissue extract when HRas pull-down was increased from 1.6 to 22 HRas per μm 2 ( g versus h ). This was not observed with the control tissue extract ( i versus j ). ( k ) Schematic of k bind inflation. Under sparse conditions of active baits on surface, a constant, single-molecule k bind is obtained even when the surface pull-down of baits is increased (left two panels). However, past the threshold at 0.6 active baits per μm 2 , more than one baits are present per ROI on average. These multiple baits have the effect of increasing k bind measured from each ROI (right panel). ( l ) k bind as a function of HRas pull-down. Error bars denote s.e. ( n >180). Full size image In an effort to describe this tumorigenesis quantitatively, we used tandem layers of antibodies; a surface-immobilized biotinylated secondary antibody and a Ras-specific primary antibody [1] , [2] . This permitted the capture of native, unlabelled Ras as well as labelled Ras ( Fig. 3c ). We first tracked Ras expression levels quantitatively through the process of tumorigenesis. Cell or tissue extracts were mixed with a diluted HEK293 cell lysate, which contained probe Ras (eGFP-HRas) of known concentration. Under the reaction conditions that fully saturate the binding sites of the primary antibody, this mixing leads to a competition for Ras-specific antibody binding between the probe Ras and target cellular Ras ( Fig. 3c , left). The number of probe Ras molecules bound to the primary antibodies falls as the concentration of target cellular Ras increases. This competitive binding decreases the number of fluorescence spots on the surface ( Fig. 3c , right), which follows the equation of when normalized to a probe Ras-only binding condition ( Supplementary Fig. S12 ). By measuring the number of bound probe molecules at several different dilutions, we were able to specifically and robustly measure the molar concentration of target cellular Ras in cell and tissue extracts ( Fig. 3d and Supplementary Fig. S12 ). This single-molecule western blot analysis indicated Ras expression levels of 42 and 59 nM in 1 mg ml −1 extracts of the cancerous MCF10A cells and xenograft tumour tissues, respectively, whereas a baseline level of 7 nM was measured in 1 mg ml −1 extracts of the control tissue ( Fig. 3e ). Furthermore, we were also able to replicate the real-time single-molecule co-IP imaging from Figs. 1 and 2 on this native Ras-capturing surface. After pulling down HRas from tumour or control tissue extracts on the tandem antibody surface, we applied a probe cell lysate, a diluted HEK293 cell lysate with 20 nM eGFP-cRaf RBD prey proteins ( Fig. 3f ). We analysed real-time co-IP traces to determine the kinetic rates k bind and k diss ( Fig. 3g–j ). It is important to note that the concentration information from the single-molecule western blot analysis ( Fig. 3e ) was crucial to ensure a specified HRas concentration for each pull down when the tumour and control tissue extracts had disparate HRas expression levels. Using the calibration data for surface pull down ( Supplementary Fig. S13 ), the concentration information was finally converted to a specific surface density of pulled-down HRas proteins ( Fig. 3g–j ). We systematically studied the change in k bind while precisely increasing the surface density of pull-down HRas proteins ( Fig. 3k ). We presume that as a result of cellular regulation, only a subset of HRas proteins on surface should be in the GTP-loaded state and show active binding events with the prey proteins. Under a sparse condition in which the distance between neighbouring active HRas molecules is far larger than the diameter of each ROI, the observed kinetics from each ROI should be independent of total HRas surface immobilization and simply report the activity of single-HRas proteins ( Fig. 3k , left two panels and Supplementary Fig. S14 ). As the surface becomes more crowded with active HRas, there should be a threshold at which there begins to be more than one active HRas molecules per ROI. Once past this threshold, the extra active HRas molecules in each ROI would produce additional fluorescence spikes that would consequently inflate k bind ( Fig. 3k , right panel and Supplementary Fig. S14 ). Indeed, we observed such biphasic trend of k bind for the tumour tissue, with a threshold at ~3 HRas pulled down per μm 2 ( Fig. 3l ). Thus, below the threshold for k bind inflation, the observed spike kinetics would largely reflect the activity of single-HRas molecules. Notably, at 1.6–1.9 HRas pulled down per μm 2 , similar k bind values of 0.28 s −1 and 0.22 s −1 were observed for the tumour and control tissue-derived HRas proteins, respectively ( Fig. 3l ). The k diss measurements were also very similar at 2.5 s −1 ( Supplementary Fig. S15 ). The tumour-derived single-oncogenic HRas consequently had an apparent dissociation constant of 180 nM, and this was very similar to the 230 nM dissociation constant for the active HRas from control tissue extract. Our observations indicate a crucial fact that the single-molecule activity of the oncogenic HRas is not dramatically different from that of an activated wild-type HRas. Then, what distinguishes this cancerous state from the normal state? The threshold for k bind inflation allows us to quantify another important statistics of cell signalling proteins, the proportion of HRas proteins actively binding with cRaf RBD . Intuitively, the threshold for k bind inflation should correspond to a specific surface density of ‘active’ bait proteins. In our imaging scheme, this threshold was found to be at 0.6 active baits per μm 2 , which does not depend on the detailed types of bait and prey proteins ( Supplementary Fig. S13 ). As the threshold for k bind inflation was observed at total 3 HRas pulled down per μm 2 , the fraction of active HRas was directly estimated to be about 20% for the tumour tissue. In contrast, we were not able to observe k bind inflation when even 25 HRas proteins were pulled down per μm 2 from the control tissue ( Fig. 3l ). These observations indicate that the oncogenic HRas derived from tumour tissue has a higher active fraction than the control tissue-derived HRas by one order of magnitude. We finally questioned whether this higher proportion of active Ras could be a simple consequence of the HRas overexpression in the xenografted tumour. The overexpressed HRas proteins could outnumber putative binding partners, left available for binding to eGFP-labelled Raf. To directly address this question, we tested two human breast cancer cell lines, MCF-7 that has wild-type KRas and MDA-MB-231 that has a mutant form of KRas (G13D; Fig. 4 ). In particular, the MDA-MB-231 cells are known to exhibit oncogene addiction to the mutated KRas gene and critically depend on aberrant KRas signalling for their survival [26] , [27] . Using these two cell lines, we are also able to determine whether our methods apply to the KRas signalling, which has pivotal importance in the molecular diagnostics and treatment of many human cancers [28] . 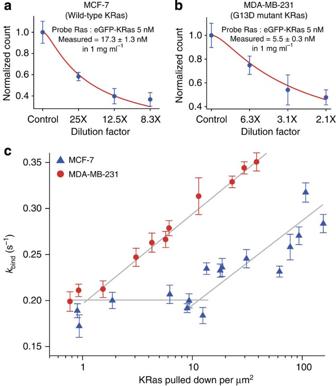Figure 4: Quantitative characterization of KRas in two human breast cancer cell lines. (a,b) Single-molecule western blot analyses of KRas expression levels. eGFP-labelled KRas was used as the probe Ras. The expression level of the wild-type KRas in the MCF-7 line was measured to be 17.3±1.3 nM, whereas that of the G13D mutant KRas in the MDA-MB-231 line was measured to be 5.5±0.3 nM per 1 mg ml−1extracts. Error bars denote s.d (n=200). (c)kbindas a function of KRas pull down. Note the samekbindvalue shared by the wild-type and mutant KRas in the single-molecule kinetics region (the common flat line). The threshold forkbindwas measured to be at 1.2 pulled down KRas per μm2for the mutant KRas from MDA-MB-231, which gave an estimated active fraction of 50%. This value was one order of magnitude higher than 6% of the wild-type KRas from MCF-7, which had the threshold at 10 KRas pulled down per μm2. Error bars denote s.e. (n>150). Figure 4: Quantitative characterization of KRas in two human breast cancer cell lines. ( a , b ) Single-molecule western blot analyses of KRas expression levels. eGFP-labelled KRas was used as the probe Ras. The expression level of the wild-type KRas in the MCF-7 line was measured to be 17.3±1.3 nM, whereas that of the G13D mutant KRas in the MDA-MB-231 line was measured to be 5.5±0.3 nM per 1 mg ml −1 extracts. Error bars denote s.d ( n =200). ( c ) k bind as a function of KRas pull down. Note the same k bind value shared by the wild-type and mutant KRas in the single-molecule kinetics region (the common flat line). The threshold for k bind was measured to be at 1.2 pulled down KRas per μm 2 for the mutant KRas from MDA-MB-231, which gave an estimated active fraction of 50%. This value was one order of magnitude higher than 6% of the wild-type KRas from MCF-7, which had the threshold at 10 KRas pulled down per μm 2 . Error bars denote s.e. ( n >150). Full size image We directly pulled down KRas from these cell extracts by using a KRas-specific primary antibody. Our single-molecule western blot analysis showed that the wild-type KRas in MCF-7 cells has a higher concentration (17 nM) than the mutant KRas in MDA-MB-231 cells (5.5 nM in 1 mg ml −1 extracts; Fig. 4a and Supplementary Fig. S16 ). Considering the KRas oncogene addiction of MDA-MB-231 cells, their smaller KRas expression level was a rather unexpected observation. Moreover, the single-molecule signalling kinetics for the wild-type and mutant KRas are essentially the same ( Fig. 4c , the common flat line; see Supplementary Fig. S15 for k diss ). On the other hand, our real-time single-molecule co-IP resolves that the threshold for k bind inflation for the mutant KRas from MDA-MB-231 is identified at 1.2 KRas pulled down per μm 2 , whereas the threshold is observed to be at ~10 KRas pulled down per μm 2 for the wild-type KRas from MCF-7 ( Fig. 4c ). As the k bind inflation always occurs at 0.6 active baits per μm 2 , these disparate thresholds directly indicate that the active fraction of the mutant KRas that strongly binds to its downstream target (15 nM cRaf RBD ) is 50%, almost one order of magnitude higher than 6% shown by the wild-type KRas. Thus, the higher active fraction exhibited by the oncogenic mutant Ras is clearly not an overexpression artefact, because the mutant KRas was expressed at lower levels, but showed a higher active fraction than the wild type. The techniques described here permit real-time imaging of co-IP processes with single-molecule resolution, which can be applied to either tagged or native proteins. We have made real-time observations of transient Ras-Raf binding events that occur in cell or tissue extracts with a half-life of hundreds of ms. Our real-time imaging has also directly visualized fast pre-equilibrating, non-specific encounter complexes, which become substrates for forming the final Ras–Raf complex. It should be noted that the time resolution and single-molecule sensitivity provided by our real-time single-molecule co-IP analysis allows us to clearly distinguish the encounter complex population from the final Ras–Raf complex. It was also recently demonstrated that through expression of eGFP-cRaf RBD , single-molecule Ras-Raf interactions could be detected in live cell fluorescence imaging [29] . Our real-time single-molecule co-IP, however, provides a general avenue for dissecting the weak, transient protein–protein interactions, which are usually invisible from conventional co-IP techniques. Simple mixing with or buffer exchange to different lysates representing various biological states will create many different situations for testing hypotheses about protein–protein interactions and cell signalling pathways. Our detection scheme for protein–protein interactions takes advantage of the difference between two time scales. Tens of μs are required for the random Brownian visits of prey proteins to the surface, but this is shorter than the duration of the Ras-Raf binding by four orders of magnitude. Using a 50-ms time resolution, only the specific Ras-Raf binding event forms a stable diffraction-limited spot on the optical fluorescence microscope. We expect the time resolution can be improved to the ms range, because it is still two orders of magnitude longer than the diffusion escape time. We might then be able to visualize very weak protein–protein interactions, including the binding of kinases to their targets. We also demonstrate that single-fluorescent proteins can be directly used as kinetic reporters for the real-time imaging of the co-IP preparation. The fact that eGFP has a roughly 80% labelling efficiency [30] and emits stable single-molecule fluorescence signals for a few seconds makes additional labelling, purification or chemical modification steps unnecessary for cell or tissue extracts. Thus, after a simple lysis step, which takes less than a hour, signalling proteins in the fresh extract can be quickly imaged and studied. Our results collectively offer key insights into the biology of Ras signalling. In particular, we have observed that the local concentration of downstream Raf proteins can be enhanced with increasing Ras surface densities. These downstream proteins are recruited in the form of encounter complexes around the Ras proteins. This encounter complex formation occurs on a far faster time scale than formation of the final Ras–Raf complex, which has the effect of enriching the downstream proteins as the substrate of the next Ras–Raf complex. Thus, we speculate that deliberate induction of a spatial association of GTP-loaded Ras proteins in the plasma membrane [31] , [32] could concentrate Raf and other downstream proteins, which in turn generates an intense signal with high temporal frequency. Single-molecule techniques [2] , [3] were mainly developed to study purified, recombinant proteins. The single-molecule co-IP techniques we are describing, however, permit a quantitative, single-molecule characterization for native protein complexes. We demonstrate, for the first time, a determination of the actively signalling fraction of Ras proteins in xenograft tumours, normal tissue and cancer cell lines. Although it is known that oncogenic Ras mutations prolong the GTP-bound state, the functional complexity of cell signalling network has made it impossible to quantify the real fraction of active, GTP-loaded Ras proteins until now. Our real-time single-molecule co-IP reveals cells tightly limit the active fraction of wild-type Ras at 5%, even in cancer cell lines. The active-Ras fraction in cancer cells carrying oncogenic Ras mutations, however, is amplified by one order of magnitude. Moreover, in the case of MDA-MB-231, this elevated active-Ras fraction leads to oncogene addiction without requiring changes in the Ras expression level or in signalling kinetics at the single-Ras level. Hence, oncogenic mutations in Ras fortify Ras signalling by taking advantage of the collective behaviour of many Ras proteins rather than producing a few individual super-active Ras proteins. Finally, we note that provided specific antibodies and fluorescently tagged prey proteins (or truncated domains) for different signalling proteins, our approaches are applicable beyond the specific Ras-Raf system we have described. This suggests a general and quantitative strategy for the characterization of signalling proteins at the level of their protein–protein interactions, which could complement genetic analyses and prove useful for precision molecular diagnostics. Gene construction and cell transfection cDNA encoding HRas (human HRas) [33] excised by EcoRI and BamHI was inserted at the C-terminus of mCherry (mCherry-C1, Clontech) or eGFP (eGFP-C1, Clontech) to generate the expression plasmids for mCherry-HRas or eGFP-HRas, respectively. The CAAX motif of HRas was deleted to prevent translocation to plasma membrane [13] . Q61L or S17N-mutated HRas was used for generating constitutively active or dominant negative HRas, respectively. For the eGFP-cRaf RBD -expression plasmid, the Ras binding domain encoding cRaf (amino acids 51–131) was inserted at the carboxy terminus of eGFP. To generate an expression plasmid for FLAG-eGFP, the FLAG tag sequence digested by NheI and AgeI and inserted at the amino terminus of eGFP (eGFP-N1, Clontech). To generate the FKBP × 2-eCFP-HRas expression plasmid, eGFP from the eGFP-HRas plasmid was replaced by enhanced cyan fluorescent protein (eCFP; Clontech) and reiterated FKBP (FKBP12) was conjugated to the N-terminus of eCFP. HEK293 and HeLa cells were obtained from American Type Culture Collection (ATCC) and maintained in Dulbecco’s modified Eagle’s medium (DMEM, Gibco) containing 10% fetal bovine serum (FBS, Gibco). For transfection, plasmid DNA was introduced into cells using a Microporator (MP-100, Digital Bio Technology). Specifically, two electric pulses of 950 V were applied to HEK293 cells for 35 ms, and two pulses of 1,000 V were applied to HeLa cells for 35 ms. Twenty-four hours after transfection, HEK293 cells were detached from the culture dish by using 0.25% Trypsin-EDTA (Invitrogen) and aliquotted into 1.5 ml tubes. Live cell co-localization study The HRas gene was tagged with eCFP and tandem FKBP domains, latter of which bind strongly to FKBP-Rapamycin Binding domain (FRB) as mediated by rapamycin. As FRB is constitutively anchored to the plasma membrane via the Lyn protein, addition of rapamycin induces translocation of FKBP × 2-eCFP-HRas to the plasma membrane. The last four residues of HRas were deleted to prevent its own plasma membrane translocation. cRaf RBD was fused to mRFP and co-expressed in the same HeLa cell. Transfected HeLa cells were aliquotted onto a 96-well glass-bottom plate (Matrical Bioscience, USA) and incubated for 24 h. Before imaging, the media was replaced with Opti-MEM Reduced-Serum Media (Invitrogen). To induce HRas translocation to the plasma membrane, cells were treated with 500 nM rapamycin (LC Laboratories) for 10 min. Multicolour and time-lapse imaging was performed on a confocal microscope (A1R, Nikon) equipped with a CFI (Nikon CFI60 Optical System). Cell and tissue lysates preparation Collected cells or tissues were dissolved in lysis buffer (150 mM NaCl, 1 mM EDTA, 1% Triton X-100, PBS) with a protease inhibitor cocktail (Sigma-Aldrich) at 4 °C for 30 min while being mixed with a pipette every 10 min. In the case of a tissue extract, frozen tissue was dissected using autopsy scissors and then mechanically grounded with electric homogenizer (T10 basic homogenizer, IKA-Werke, GMBH) in PBS on ice supplemented with 1% Triton X-100, 1 μg ml −1 pepstatin A, 1 μg ml −1 leupeptin, 1 mM phenylmethanesulfonylfluoride, 1 mM sodium fluoride and 1 mM sodium orthovanadate. This lysate was centrifuged at 12,000 g for 10 min and the supernatant was collected. Bio-Beads SM-2 (Bio-Rad) were washed three times with methanol and then five times with deionized water. A measure of 50 mg of cleaned beads were used per 300 μl lysate and this mixture was rotated at 4 °C for 2 h. Beads were finally removed, and the solution was used for single-molecule experiments. Recombinant eGFP (BioVision) and mCherry (BioVision) were used to determine the concentrations of fluorescently tagged proteins in the cell lysates. The fluorescence levels for recombinant eGFP and mCherry proteins of known concentrations (5 to 25 nM, at least five different concentration points) were measured using a fluorometer (Enspire 2300, Perkin-Elmer) and used to make a calibration curve. Cell lysates were diluted by a proper factor such that the concentrations of expressed proteins could be determined using the calibration curve from the recombinant protein. We used the DC protein assay kit (Bio-Rad) to measure the total protein concentration of a cell lysate. Real-time single-molecule co-IP imaging A quartz slide was cleaned using piranha solution and then coated with 100:1 (mol/mol) methoxypolyethylene glycol (mPEG):biotin-PEG (Laysan Bio). This PEG-coated surface was placed on the bottom surface of a microfluidic chamber [34] . A layer of neutravidin (Invitrogen) was formed via a 5-min incubation at 1.6 μM. Biotinlyated antibodies targeting mCherry (ab34771, Abcam) or FLAG (F9291, Sigma-Aldrich) were directly immobilized on the neutravidin layer to selectively capture mCherry-HRas and FLAG-eGFP, respectively. To form the tandem antibody layers for pulling down native HRas or KRas proteins, we used biotinylated secondary antibodies for rabbit (Biotin-conjugated goat anti-rabbit IgG, Fc fragment specific, 111-065-046, Jackson Immuno Reaserch) and anti-HRas primary antibodies (SC-520, Santa Cruz) or anti-KRas primary antibodies (SC-521, Santa Cruz). For surface immobilization of bait proteins, the cell extracts were directly applied to this antibody-immobilized surface through microfluidic buffer exchange. After a 5-min incubation, the first cell extract was removed by buffer exchange with PBS. The microfluidic chamber was then placed on a prism-type TIRF microscope (customized IX-71, Olympus), with the quartz surface used as the imaging plane ( Fig. 1c ). For the real-time imaging of single-molecule co-IP, a second cell extract containing eGFP-tagged prey proteins was injected at 50 μl s −1 using a syringe pump (KD Scientific), while an electron-multiplying charge-coupled device (EM-CCD; iXon DU897v, Andor Technology) recorded real-time movies with 50 ms time resolution. A dichroic mirror with its threshold at 580 nm (Chroma) separated the collected fluorescence signals into two rays, and the customized dual-view setup formed two images of the imaging area (45 × 90 μm 2 ) on the EM-CCD chip (256 × 512 pixels used without binning for each image). These two images are denoted the eGFP (below 580 nm) and mCherry (above 580 nm) channels, respectively. ROI 7 pixels in diameter (corresponding to an area of 1.1 μm 2 ) were designated by a computer algorithm (written in IDL, ITT Visual Information Solutions) that averaged every ten frames from the TIRF images and selected local Gaussian maxima. A real-time trace of fluorescence signal was generated from each ROI using scripts written in MATLAB. Transformation to cancerous cells and orthotopic xenograft MCF10A cells were grown in DMEM/F12 supplemented with 5% horse serum, 20 ng ml −1 epidermal growth factor, 0.5 μg ml −1 hydrocortisone, 10 μg ml −1 insulin, 100 ng ml −1 cholera toxin and penicillin/streptomycin. MCF-7 and MDA-MB231 cells were grown in DMEM supplemented with 10% FBS and antibiotics. To generate MCF10A cells with constitutively active HRas, HEK293T cells in DMEM supplemented with 10% FBS and penicillin/streptomycin were co-transfected with pMSCV Neo HRas(G12V), pGP (encoding MuLV Gag-Pol) and pVpack-VSV-G (Stratagene) with polyethyleneimine (PEI, Polyscience). Forty-eight hours after transfection, the culture supernatant containing viral particles was collected and centrifuged to clear cell debris. These viral particles, diluted in 1:5 ratio with MCF10A media supplemented with 6 μg ml −1 polybrene (Sigma), were applied to MCF10A. A total of 2 × 10 6 MCF10A HRas(G12V) cells were resuspended in 100 μl of PBS with 50% growth factor reduced Matrigel (BD Biosciences). The cell suspensions were injected into the mammary fat pad of 5-week-old female nude mice (BALB/c, Charles River Lab). The mice were killed 17 days after the xenograft, and the tumour was taken out and snap frozen with liquid nitrogen for later analyses. Single-molecule western blot analysis A monoclonal primary antibody (ab52939, Abcam) was used because of its faster binding to Ras proteins. This primary antibody, however, would be difficult to be used for real-time co-IP imaging because its binding site includes the active site of Ras. A cell or tissue extract with unknown HRas (or KRas) concentration was serially diluted by different factors, and each dilution was mixed with eGFP-HRas (or eGFP-KRas) of a known concentration (nM to tens of nM used for the probe Ras) and primary antibody diluted 16,700-fold ( Supplementary Fig. S12 ). Glutaraldehyde at a concentration of 0.05% was added as a cross-linker to the binding reaction. We have confirmed that the cross-linker was neither autofluorescent nor did it induce non-specific surface binding of the probe Ras. One hour with the cross-linker was long enough to saturate the binding reaction for the monoclonal anti-Ras antibody used in this work. Each solution was then incubated on a surface coated with secondary antibody to immobilize the primary antibodies saturated with cellular and probe proteins. This incubation time can be adjusted such that the number of sampled primary antibody molecules is appropriate for single-molecule counting (that is, roughly 500–800 molecules per imaging area). We used 800 primary antibody molecules ( N total ) per imaging area ( Supplementary Fig. S12 ). Our scheme minimizes the incubation time of tissue extracts on the surface to reduce autofluorescence ( Supplementary Fig. S12 ). After microfluidic buffer exchange to PBS, we counted the number of fluorescence spots per imaging area ( N fluor ) using the TIRF microscope. N fluor was measured for several dilution factors. Finally, the cellular Ras concentration ([Ras]) was calculated by fitting the curve to the equation, , where α −1 is the dilution factor. The square term is needed because each primary antibody binds to two HRas proteins. How to cite this article: Lee, H.-W. et al. Real-time single-molecule co-immunoprecipitation analyses reveal cancer-specific Ras signalling dynamics. Nat. Commun. 4:1505 doi: 10.1038/ncomms2507 (2013).